Plant species determine tidal wetland methane response to sea level rise Blue carbon (C) ecosystems are among the most effective C sinks of the biosphere, but methane (CH 4 ) emissions can offset their climate cooling effect. Drivers of CH 4 emissions from blue C ecosystems and effects of global change are poorly understood. Here we test for the effects of sea level rise (SLR) and its interactions with elevated atmospheric CO 2 , eutrophication, and plant community composition on CH 4 emissions from an estuarine tidal wetland. Changes in CH 4 emissions with SLR are primarily mediated by shifts in plant community composition and associated plant traits that determine both the direction and magnitude of SLR effects on CH 4 emissions. We furthermore show strong stimulation of CH 4 emissions by elevated atmospheric CO 2 , whereas effects of eutrophication are not significant. Overall, our findings demonstrate a high sensitivity of CH 4 emissions to global change with important implications for modeling greenhouse-gas dynamics of blue C ecosystems. Tidal wetlands (i.e. marshes and mangroves) are often characterized by lower emissions of the powerful greenhouse gas CH 4 than nontidal wetlands [1] , [2] , [3] , [4] . Microbial CH 4 production in wetland soils is governed by the balance of electron donors and terminal electron acceptors [5] . Lower CH 4 emissions in tidal vs. nontidal wetlands result from higher soil concentrations of sulfate, which acts as a terminal electron acceptor and allows sulfate-reducing bacteria to outcompete methanogenic communities for electron donors [5] , [6] . Site salinity, a proxy for sulfate availability, is the best-established predictor of CH 4 emissions from tidal wetlands, but it weakly constrains emission rates [6] , [7] . Overall, CH 4 emissions from tidal wetlands are extremely variable, and many sites emit CH 4 at rates that exceed C sequestration in terms of CO 2 equivalents [2] , [8] , [9] . Drivers of variability in CH 4 emissions other than sulfate are poorly understood [7] , [10] . Only few case studies have elucidated other important drivers of CH 4 emissions, such as sedimentation dynamics [11] , organic matter quality and quantity [7] , tidal pumping [12] , and functional trait composition of plant communities [13] , [14] , [15] . Therefore, the consequences of perturbations on radiative forcing from tidal wetlands are difficult to predict and often unknown, currently representing one of the biggest challenges in blue C science [16] . Global change alters C sequestration and greenhouse-gas dynamics across ecosystems. In tidal wetlands, accelerated relative sea level rise (SLR) represents the overriding global change factor affecting ecosystem function in the long-term [17] , [18] , [19] . Although SLR poses a major threat to the stability of tidal wetlands, it also enhances their C stocks globally by stimulating C sequestration in soils [18] , [20] . SLR effects on tidal wetlands can therefore induce an important negative feedback to global warming [20] . Conversely, as SLR increases flooding frequency, leading to increasingly anaerobic soil conditions, it also yields the potential to stimulate CH 4 emissions. It is therefore possible that SLR-stimulated soil C sequestration is offset or even reversed by SLR stimulation of CH 4 emissions. Methane emissions from nontidal wetland ecosystems often increase in response to global change factors such as elevated atmospheric levels of CO 2 , rising temperatures, and eutrophication [21] , [22] , [23] , [24] , [25] . Stimulated CH 4 emissions in response to global change are often driven by the strong control of plant processes on soil CH 4 dynamics. Plants can stimulate CH 4 emissions from soils by increasing the input of organic matter serving as electron donors. Particularly, the input of recent photo-assimilates to the soil via root exudation is known to fuel methanogenic communities [5] , [26] . However, it is unclear if CH 4 responses to commonly studied global change factors in nontidal wetlands are transferable to tidal wetlands where SLR strongly interacts and often dominates other global change factors, modulating their effects on plant traits and microbial processes such as primary production and decomposition [18] , [27] , [28] . We therefore argue that the overriding control of SLR on tidal wetland functioning needs to be considered when estimating the effects of other global change drivers on CH 4 emissions. The effects of SLR on CH 4 emissions and the degree to which SLR modulates the effects of other global changes on CH 4 emissions has never been studied and cannot easily be projected. For instance, SLR-induced increases in flooding frequency are likely to exert opposing effects on the availability of two terminal electron acceptors that suppress methanogenesis, namely sulfate and oxygen. In addition, the relationship between sea level and electron donor availability (i.e. plant productivity) is not linear [29] , [30] , further complicating projections of CH 4 dynamics in tidal wetlands. Here we investigate the effects of SLR and its interactions with elevated atmospheric CO 2 and coastal eutrophication (i.e. elevated nitrogen levels) on CH 4 emissions from an estuarine tidal wetland. Multifactorial manipulations were implemented by applying a unique experimental design that combines field-deployed marsh mesocosms for sea level manipulation [31] and floating open top chambers to control atmospheric CO 2 concentrations [27] . Relationships observed in mesocosm studies were then tested against field data. We hypothesized that CH 4 emissions would increase in response to all factors—SLR, elevated CO 2 , and eutrophication—and that SLR would be the dominant factor because of the strong control it exerts on oxygen availability. We predicted that CH 4 emissions would rise monotonically with SLR, and be greater within a given sea level when CO 2 or nitrogen were added as resources. We observed increases in CH 4 emissions in response to SLR and elevated CO 2 , but not to eutrophication. SLR indeed exerted the strongest control on CH 4 emissions; however, its effect was nonlinear rather than monotonic, initially decreasing with SLR before increasing with SLR. This unexpected pattern in CH 4 emissions was primarily mediated by SLR-driven shifts in plant community composition that determined both the direction and magnitude of the CH 4 response. Subsequent in-situ observations confirmed that the same pattern occurs at the field-plot scale. Our findings therefore demonstrate that predictions of current and future greenhouse-gas dynamics of blue C ecosystems will require understanding of plant community dynamics and traits relevant to CH 4 cycling. Multiple global change effects on CH 4 emissions Global change treatments (sea level × nitrogen fertilization × elevated CO 2 ) were applied in a full-factorial design, and effects were analyzed using three-way (split plot) ANOVA [27] (Experiment 1). 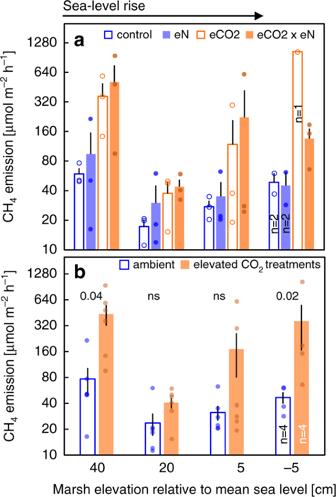Fig. 1: Interacting global change effects on CH4emissions. aCH4emissions from field-based mesocosms of Experiment 1 exposed to four different sea level treatments (elevations relative to mean sea level) and full-factorial manipulations of nitrogen and CO2availability. (control = ambient nitrogen and ambient CO2; eN = elevated nitrogen and ambient CO2; eCO2= elevated CO2and ambient nitrogen; eCO2× eN = elevated CO2and elevated nitrogen). Data are presented as means ± SEM (n= 3 experimental units per group, based on mean values of duplicate mesocosms) and all datapoints are overlaid. Divergences from replication result from plant die-off at low elevations and are specified.bAmbient vs. elevated CO2treatments pooled for clearer illustration of eCO2effects.Pvalues above bars denote significant main effects (p≤ 0.05) of the CO2treatment on CH4emissions (two-way ANOVA for each elevation separately). Data are presented as means ± SEM (n= 6 per group), divergences from replication are specified. The fraction of time flooded varied across the four sea level treatments as follows: 3–22–53–74%. Elevated CO2treatments were exposed to ambient [CO2] + 300 ppm. Elevated N treatments received 25 g N m−2on a biweekly basis. Sea level manipulations exerted the strongest effect on CH 4 emissions ( F = 10.78; p ≤ 0.001; Table 1 ; Fig. 1 ). The effect of relative sea level was nonlinear, counter to the expectation that increasing flooding will monotonically increase CH 4 emissions. CH 4 emissions were greatest at +40 cm above mean sea level (MSL; least-flooded elevation), show a steep drop from +40 cm to +20 cm above MSL, then increase from +20 cm to –5 cm (most-flooded elevation). Emissions from the least- and most-flooded elevations were not significantly different (Fig. 2a ). Nonlinear regression analysis suggests a unimodal relationship between sea level and CH 4 emissions (log CH 4 emissions (MSL) = 0.001 x 2 − 0.04 x + 1.78; R 2 = 0.30; p ≤ 0.001; Supplementary Fig. 1 ). Table 1 Results of three-way split-plot ANOVA testing for effects of sea level, CO 2 , and nitrogen treatments on CH 4 emissions ( n = 3). Full size table Fig. 1: Interacting global change effects on CH 4 emissions. a CH 4 emissions from field-based mesocosms of Experiment 1 exposed to four different sea level treatments (elevations relative to mean sea level) and full-factorial manipulations of nitrogen and CO 2 availability. (control = ambient nitrogen and ambient CO 2 ; eN = elevated nitrogen and ambient CO 2 ; eCO 2 = elevated CO 2 and ambient nitrogen; eCO 2 × eN = elevated CO 2 and elevated nitrogen). Data are presented as means ± SEM ( n = 3 experimental units per group, based on mean values of duplicate mesocosms) and all datapoints are overlaid. Divergences from replication result from plant die-off at low elevations and are specified. b Ambient vs. elevated CO 2 treatments pooled for clearer illustration of eCO 2 effects. P values above bars denote significant main effects ( p ≤ 0.05) of the CO 2 treatment on CH 4 emissions (two-way ANOVA for each elevation separately). Data are presented as means ± SEM ( n = 6 per group), divergences from replication are specified. The fraction of time flooded varied across the four sea level treatments as follows: 3–22–53–74%. Elevated CO 2 treatments were exposed to ambient [CO 2 ] + 300 ppm. Elevated N treatments received 25 g N m −2 on a biweekly basis. Full size image Fig. 2: Plant species control on CH 4 emissions and soil redox. a CH 4 emissions and b aboveground biomass of Experiment 1 mesocosms exposed to four different sea level treatments (elevations relative to mean sea level); all CO 2 - and nitrogen-treatment combinations are pooled ( n = 12 experimental units per group, based on means of duplicate mesocosms). Field-based mesocosms were planted with mixed communities of Schoenoplectus americanus and Spartina patens . c CH 4 emissions and d soil redox conditions (10 cm soil depth) of Experiment 2 mesocosms. Field-based mesocosms were either planted with Schoenoplectus americanus or Spartina patens and exposed to two different sea level treatments. CH 4 emissions were measured on n = 4 and redox on n = 3 mesocosms per group. All panels show means ± SEM plus an overlay of single datapoints. P values in a denote significant differences ( p ≤ 0.05) based on Tukey’s HSD test. Two-way ANOVA results are shown in c , d . Data in b are redrawn after Langley et al. [27] . Data from Schoenoplectus -planted mesocosms in c , d are taken from Mueller et al. [50] . Full size image The nitrogen fertilization treatment and any interactions thereof did not affect CH 4 emissions (all F values ≤ 0.65; all p values ≥ 0.59; Table 1 ; Fig. 1a ). By contrast, an apparent CO 2 effect was indicated ( F = 5.84; p = 0.07; Table 1 ), but likely masked to a certain degree by the overriding effect of the sea level treatment on our results. Indeed, two-way analyses within sea level treatments confirmed significant and strong stimulation of CH 4 emissions by elevated CO 2 , with mean stimulation ranging from 70% at +20 cm to 670% at −5 cm relative to MSL (Fig. 1b ). Species shifts control global change effects on CH 4 emissions Experiment 1 was designed to examine the effects of interacting global change factors on plant growth in the context of interspecific competition [27] , and therefore global change treatments were applied to realistic plant assemblages, not single species. Plant responses of the two dominant species, the C4 grass Spartina patens (hereafter Spartina ) and the C3 sedge Schoenoplectus americanus (hereafter Schoenoplectus ), to sea level treatments reflected their abundance and biomass allocation along the natural elevation gradient and the SLR-driven encroachment of flooding tolerant Schoenoplectus into Spartina communities of the adjacent reference marsh and elsewhere [27] , [29] , [32] , [33] , [34] (Fig. 2b , compare Langley et al. [27] for a detailed presentation of plant biomass responses). Here we found an unforeseen sharp decrease in CH 4 emissions with rising sea level in the higher parts of the tidal frame (Fig. 2a ). This result was unexpected, because soil oxygen availability should have decreased as flooding duration increased from high to low elevations [27] , [35] , simultaneously enhancing methanogenesis and suppressing methanotrophy. In the following we argue that the observed decrease in CH 4 emissions was driven by a shift in species dominance from Spartina , dominant at high elevations of the marsh, to Schoenoplectus , dominant at low elevations (Fig. 2b ). CH 4 emissions were inversely related to Schoenoplectus aboveground biomass across all treatment combinations (log CH 4 emissions = −0.0004 x + 2.307; R 2 = 0.144; p ≤ 0.01). Relationships between biomass parameters and CH 4 emissions were much stronger when restricted to certain CO 2 - and nitrogen-treatment combinations. Specifically, CH 4 emissions showed the strongest negative relation to Schoenoplectus aboveground biomass within ambient CO 2 -treatment combinations (Fig. 3 ), although similar but weaker relationships were also found under elevated CO 2 (Supplementary Fig. 2 ). The opposite response was observed in relation to Spartina aboveground biomass, which scaled positively with CH 4 emissions under ambient CO 2 (Fig. 3 ). Relationships between biomass parameters and CH 4 emissions were strongest when the dataset was restricted to the highest (least flooded) two treatments (+40 cm and +20 cm above MSL; Fig. 3 ), where changes in CH 4 emissions were most pronounced (Fig. 2a ) and dominance of the two species was most balanced (Fig. 2b ). Relationships of CH 4 emissions with plant parameters other than aboveground biomass were not significant, neither across nor within treatment groups (Supplementary Tables 1 and 2 ). Fig. 3: CH 4 emissions as function of aboveground biomass parameters. Relationships between aboveground biomass and log CH 4 emissions within ambient CO 2 treatments of Experiment 1. a – c Relationships across all four sea level treatments ( n = 32 mesocosms) and d – f across the two highest (least flooded) treatments (+40 cm and +20 cm above mean sea level; n = 20 mesocosms). Linear regression is shown for significant relationships ( p ≤ 0.05). Biomass data are taken from Langley et al. [27] . Full size image Plot-scale CH 4 data from the adjacent Smithsonian Global Change Research Wetland (GCReW) support the mesocosm results. Mean growing season CH 4 emissions were strongly related to the relative abundance of the two species (Fig. 4 ) and over three times greater from the higher elevation Spartina -dominated community of the marsh (65 ± 37 µmol m −2 h −1 ) than from the lower elevation Schoenoplectus -dominated community (20 ± 5 µmol m −2 h −1 ; p ≤ 0.05; n = 3). Both absolute CH 4 emission rates and differences induced by community composition correspond well to the findings of Experiment 1 (Fig. 1a , control treatment). Fig. 4: CH 4 emissions from field plots. In-situ CH 4 emissions as a function of the aboveground biomass contributed by the C3 sedge Schoenoplectus americanus relative to total aboveground biomass, the remainder of which was C4 grasses ( Spartina patens with small contributions of Distichlis spicata ). CH 4 data are means of monthly in-situ flux measurements conducted during the 2019 growing season (Jun–Sep) across all ambient CO 2 plots of the Salt Marsh Accretion Response to Temperature eXperiment (SMARTX) ( n = 24 field plots). Full size image In order to evaluate the importance of these plant species-specific effects in mediating the relationship between sea level and CH 4 emissions in the upper tidal frame, a follow-up marsh organ experiment was conducted (Experiment 2). Experiment 2 did not use mixed species assemblages as in Experiment 1, but instead used pure communities of Schoenoplectus or Spartina to isolate species-level effects at two different sea levels. CH 4 emissions between the two species were dramatically different. Mean CH 4 emissions were 55 and 65 times greater from Spartina compared to Schoenoplectus at +15 cm and +35 cm above MSL, respectively ( F = 40.80; p ≤ 0.001; Fig. 2c ). Sea level ( F = 1.43; p = 0.26) and the interaction of sea level and plant species ( F = 0.20; p = 0.66) did not affect CH 4 emissions (Fig. 2c ) demonstrating that CH 4 emissions as a function of sea level are primarily mediated by shifts in plant species composition, and that the direct (i.e. non-plant mediated) control of sea level on electron acceptor availability, such as oxygen, iron, and sulfate, is of less importance. In contrast to the clear effects of sea level on Spartina vs. Schoenoplectus dominance in Experiment 1, CO 2 and nitrogen treatments did not induce significant shifts in species dominance within the mixed communities [27] , demonstrating the stronger control of sea level than other global change factors on species composition. Both CO 2 and nitrogen treatments produced positive effects on plant biomass [27] , but these did not translate into changes in CH 4 emissions. Nitrogen fertilization strongly and consistently increased Schoenoplectus and Spartina biomass across elevations [27] but had no effect on CH 4 emissions (Table 1 and Fig. 1a ). Elevated CO 2 significantly increased Schoenoplectus and total aboveground biomass [27] , two factors that were negatively related to CH 4 emissions (Fig. 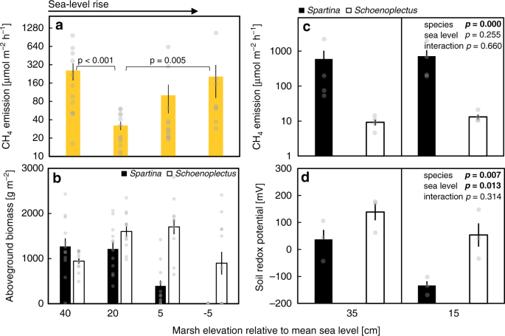Fig. 2: Plant species control on CH4emissions and soil redox. aCH4emissions andbaboveground biomass of Experiment 1 mesocosms exposed to four different sea level treatments (elevations relative to mean sea level); all CO2- and nitrogen-treatment combinations are pooled (n= 12 experimental units per group, based on means of duplicate mesocosms). Field-based mesocosms were planted with mixed communities ofSchoenoplectus americanusandSpartina patens.cCH4emissions anddsoil redox conditions (10 cm soil depth) of Experiment 2 mesocosms. Field-based mesocosms were either planted withSchoenoplectus americanusorSpartina patensand exposed to two different sea level treatments. CH4emissions were measured onn= 4 and redox onn= 3 mesocosms per group. All panels show means ± SEM plus an overlay of single datapoints.Pvalues inadenote significant differences (p≤ 0.05) based on Tukey’s HSD test. Two-way ANOVA results are shown inc,d. Data inbare redrawn after Langley et al.27. Data fromSchoenoplectus-planted mesocosms inc,dare taken from Mueller et al.50. 3 and Supplementary Table 2 ), implying that the strong and positive effect of elevated CO 2 on CH 4 emissions (Fig. 1 ) was driven by plant processes that are not directly linked to biomass. One likely process is the well-documented phenomenon of increased root exudation in response to elevated CO 2 [36] , [37] , [38] , [39] , acting as primary energy source for methanogenic communities [5] . In accordance with our findings, data from a long-term elevated CO 2 experiment in the adjacent GCReW field site show a strong CO 2 stimulation of CH 4 emissions from pure stands of Schoenoplectus [40] . Furthermore, elevated CO 2 increased both porewater concentrations of CH 4 and dissolved organic C [41] , effects that could likewise be attributed to greater inputs of organic matter via root exudation or rapid root turnover. Previous work conducted at larger plot scales and over multiple years in mixed communities of the GCReW site has shown that elevated CO 2 and nitrogen fertilization shift the balance between Schoenoplectus and Spartina in opposite directions (i.e. nitrogen favored Spartina over Schoenoplectus and vice versa) [42] . Given the overriding control of plant community composition on CH 4 emissions found in the present study, this implies that the longer-term effects of these global change factors may differ from the effects presented here, which reflect relatively short-term effects over two growing seasons. However, the present work also demonstrates that SLR represents an overriding global change driver in the studied system. We therefore argue that shifts in plant species dominance in response to elevated CO 2 and nitrogen fertilization observed under ambient rates of SLR [42] , [43] may be less important under higher rates of SLR as simulated in the present study. This notion is supported by the observation that decadal‐scale oscillations in local sea level at GCReW have stronger effects on plant community composition than elevated CO 2 and nitrogen fertilization treatments of the long-term field experiments [34] , [44] . 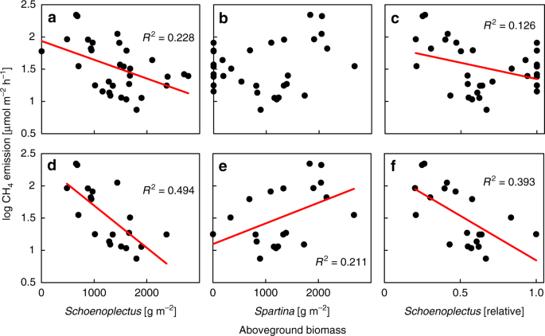Fig. 3: CH4emissions as function of aboveground biomass parameters. Relationships between aboveground biomass and log CH4emissions within ambient CO2treatments of Experiment 1.a–cRelationships across all four sea level treatments (n= 32 mesocosms) andd–facross the two highest (least flooded) treatments (+40 cm and +20 cm above mean sea level;n= 20 mesocosms). Linear regression is shown for significant relationships (p≤ 0.05). Biomass data are taken from Langley et al.27. 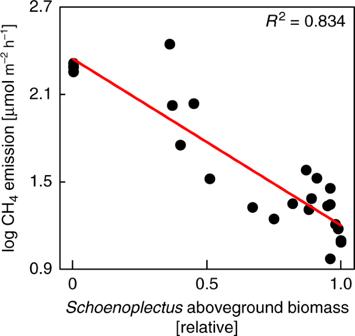Fig. 4: CH4emissions from field plots. In-situ CH4emissions as a function of the aboveground biomass contributed by the C3 sedgeSchoenoplectus americanusrelative to total aboveground biomass, the remainder of which was C4 grasses (Spartina patenswith small contributions ofDistichlis spicata). CH4data are means of monthly in-situ flux measurements conducted during the 2019 growing season (Jun–Sep) across all ambient CO2plots of theSalt Marsh Accretion Response to Temperature eXperiment(SMARTX) (n= 24 field plots). Plant traits affecting CH 4 dynamics In accordance with clear plant species effects on CH 4 emissions, soil redox conditions in the pure communities of Experiment 2 were more strongly affected by plant species than by sea level (Fig. 2d ). Redox was markedly higher in Schoenoplectus vs. Spartina rhizospheres by c. 180 and 100 mV at +15 and +35 cm above MSL, respectively ( F = 13.0; p ≤ 0.01). Soil redox conditions reflect the balance between plant-mediated transport of electron donors and acceptors. Therefore, our findings demonstrate either a greater provision of electron acceptors (i.e. oxygen) or a lower provision of electron donors (organic matter) in Schoenoplectus vs. Spartina rhizospheres. Importantly, both mechanisms would cause lower CH 4 production in Schoenoplectus rhizospheres. Redox was significantly higher at +35 cm above MSL than at the lower and more frequently flooded +15 cm treatment ( F = 10.2; p ≤ 0.05), demonstrating the expected suppression of rising sea level on oxygen availability. Notably, there was no statistical difference ( p = 0.99) in soil redox potential in the presence of Schoenoplectus at the wettest treatment (+15 cm) and Spartina at the driest (+35 cm) treatment (Fig. 2d ). Consistent with our CH 4 results, this demonstrates a stronger plant vs. sea level control on soil redox conditions in the studied system and underpins the primary control of plant species composition, and to a lesser degree sea level per se, on soil biogeochemistry. The redox data suggest that greater CH 4 emissions in Spartina vs. Schoenoplectus are driven by plant traits affecting the balance between plant-mediated transport of electron donors and acceptors into the soil. There is abundant evidence to support greater supply of oxygen to the rhizosphere by Schoenoplectus vs. Spartina via root oxygen loss. Studies conducted on morphologically similar species of the same genus in tidal freshwater and nontidal wetland systems demonstrated markedly higher plant-stimulation of oxidation than production of CH 4 [13] , [45] , [46] , [47] . Root oxygen loss by wetland plants supports higher rates of CH 4 oxidation and stimulates the decomposition of soil organic matter, a phenomenon called priming [48] . Previous work at the study site demonstrated high rates of priming in Schoenoplectus rhizospheres, whereas priming in Spartina rhizospheres was absent or even negative [49] . This finding provides further evidence of higher oxygen transport to soils by Schoenoplectus than Spartina , and it suggests opposing effects of root oxygen loss on priming and CH 4 emissions in a greenhouse-gas context. Indeed, in a past study we also demonstrated that priming in Schoenoplectus rhizospheres scales positively with aboveground biomass [50] , opposite the response of CH 4 emissions to aboveground biomass in the present study (Fig. 3a, d ). The contrasting effects of the two species on CH 4 emissions may also be caused by differences in electron donor input, such as higher rates of root exudation in Spartina vs. Schoenoplectus rhizospheres. Recent studies in Chinese tidal wetlands demonstrated that invasive Spartina alterniflora stimulated CH 4 emissions through higher exudation of labile organic substrates from S. alterniflora roots in comparison to native species [15] , [51] . We do not have data on root exudate quality and quantity in Spartina - vs. Schoenoplectus -dominated mesocosms, but data from the adjacent reference marsh platform indeed show markedly higher porewater concentrations of dissolved organic C in Spartina [41] , [52] . One alternative explanation for greater CH 4 emissions from Spartina vs. Schoenoplectus is that Spartina supports greater rates of plant transport of CH 4 from the soil via the plant-aerenchyma system. This explanation, however, is implausible because Spartina patens has a poorly developed aerenchyma system compared to Schoenoplectus americanus [53] , and concentrations of porewater CH 4 in the adjacent reference marsh are higher in Spartina vs. Schoenoplectus rhizospheres [52] . Taken together, it is likely that two processes—higher root oxygen loss by Schoenoplectus and higher root exudation by Spartina —explain the contrasting effects of these species on CH 4 emissions in the present study and thereby determined the dramatic change in CH 4 emissions in response to sea level-induced species shifts. Implications Other than salinity, drivers of variability in CH 4 emissions from tidal wetlands are poorly understood, which represents one of the biggest challenges to building robust numerical forecast models of greenhouse-gas dynamics for blue C ecosystems [16] . CH 4 emissions from the ambient CO 2 treatments of our main experiment ranged between 2.3 and 8.4 g CH 4 m −2 year −1 (Fig. 1b ) and thereby reflect the lower spectrum of reported values for mesohaline marshes based on a recent global meta-analysis (−0.5 to 551.1 g CH 4 m −2 year − 1 ) [7] and earlier work with focus on North America (3.3–32.0 g CH 4 m −2 year −1 ) [6] . Relative sea level exerted a strong, nonlinear control on CH 4 emissions. The difference between lowest and highest mean CH 4 emissions was 31 g CH 4 m −2 year −1 (Fig. 2a ), corresponding to c. 6% of the total range of CH 4 emissions reported for tidal marshes globally [7] and to c. 95% of the total range reported for differences between meso- and polyhaline tidal marshes based on the salinity-CH 4 model of Poffenbarger et al. [6] . We furthermore show strong positive effects of elevated CO 2 which increased CH 4 emissions an amount similar to sea level effects. Our study thereby identifies two important drivers of CH 4 emissions both with a large potential to change the future greenhouse-gas balance of blue C ecosystems. The main value of the present work is based on the mechanisms it illustrates, which are largely independent of absolute effect sizes. This is the first study to experimentally test if SLR interacts with other global change factors to change CH 4 emissions from blue C ecosystems. We demonstrate that predictions of both direction and magnitude of sea level effects on CH 4 emissions require an understanding of plant species traits that have the capacity to drive dramatic changes in redox chemistry. Furthermore, we show that effects of the global change factors elevated CO 2 and nitrogen interact differently with sea level. Effects of nitrogen fertilization were consistently null while the effects of elevated CO 2 were consistently positive. Indeed, CO 2 effects tended to amplify with more extreme sea levels. Our findings therefore yield important implications for modeling current and future greenhouse-gas dynamics of blue C ecosystems. Study site The study was carried out in a tidal wetland site on Rhode river, a sub-estuary of the Chesapeake Bay in Maryland, USA (38°53′N, 76°33′W). The field site is home to the GCReW site operated by the Smithsonian Environmental Research Center. Tidal amplitude at the site is <50 cm and salinity generally <15 ppt. Soils are peats with organic matter contents >80%. Site vegetation is dominated by the C3 sedge Schoenoplectus americanus (hereafter Schoenoplectus ) at lower, more frequently flooded elevations and by the C4 grass Spartina patens (hereafter Spartina ) at higher, less frequently flooded elevations. The two species occur in pure and mixed communities depending on surface elevation. Over the past two decades, a fast, SLR-driven encroachment of Schoenoplectus into Spartina communities has been observed [34] . Plant growth at the site is nitrogen limited. Ammonium makes up >99% of the porewater inorganic nitrogen pool, and nitrate concentrations are usually below detection limits [42] , [54] . The main tidal creek of the GCReW site accommodates a marsh organ facility. Marsh organs ( sensu Morris [31] ) consist of field-based mesocosms arranged at different elevations, and thus different relative sea levels, to manipulate flooding frequency and assess the effects of accelerated relative SLR on plant and soil processes. Here we report on the results of two separate marsh organ experiments conducted between 2011 and 2012. Experimental designs The design of Experiment 1 has been described by Langley et al. [27] and was originally designed to study the effects of interacting global change factors on plant growth. It represents the first study to combine marsh organs and open top chambers to manipulate relative sea level and atmospheric CO 2 concentrations at the same time. An additional component of the study is an elevated nitrogen treatment. The three treatments were applied in a full-factorial design. Mesocosms (70-cm deep, 10-cm diameter) were filled with peat soil, planted with mixed native species assemblages of Spartina and Schoenoplectus , and evenly distributed on six separate marsh organs ( n = 24 per marsh organ). Initial planting reflected natural stem densities of the two species in the adjacent high mash [27] . Within each marsh organ, mesocosms were installed at the following six elevations in relation to MSL of the growing season (May–Sep): MSL −25 cm, MSL −15 cm, MSL −5 cm, MSL +5 cm, MSL +20 cm, and MSL +40 cm. Treatments covered the current relative sea level range of the adjacent marsh (three highest elevations) as well as future sea level scenarios (three lowest elevations) [27] , [54] . Long-term average SLR (90-year trend) at the site is c. 4 mm year −1 . MSL was calculated based on tide gauge data (Annapolis, MD, Station ID: 8575512, URL: https://tidesandcurrents.noaa.gov ) after each growing season and could therefore only be estimated before mesocosm deployment. The fraction of time flooded ranged from 3% to 96% across the six elevations [27] . The elevated CO 2 treatment was applied by placing a floating open top chamber over each of the six marsh organs that was capable of rising and falling with the tide cycle. Three of the marsh organs were exposed to elevated CO 2 (ambient [CO 2 ] + 300 ppm, simulating an atmospheric CO 2 scenario projected for the year 2100 [55] ) by receiving additional CO 2 mixed into the air stream of a blower system connected to each open top chamber. The other three marsh organs were equipped with identical open top chambers and air blower systems but did not receive additional CO 2 via the air stream. Half of the mesocosms were exposed to an elevated nitrogen treatment projected to increase soil mineral nitrogen concentrations by c. 40%. Ammonium chloride solution equivalent to an nitrogen input of 25 g N m −2 was injected to the rhizosphere on a biweekly basis throughout the growing season. A follow-up marsh organ experiment, Experiment 2, was conducted to separate effects of plant species identity (i.e. Schoenoplectus vs. Spartina ) from effects of interspecific plant competition on CH 4 emissions. This experiment used monocultures of either Schoenoplectus or Spartina , and no CO 2 or nitrogen treatments were applied. Mesocosms were exposed to three sea level treatments: MSL ±0 cm, MSL +15 cm, and MSL +35 cm. For details we refer the reader to Mueller et al. [50] . Mesocosm artifacts need to be considered when interpreting the absolute rates of CH 4 emissions and effect sizes reported here. For instance, marsh organ experiments at GCReW, including the present experiments, generally produce more biomass per area than the adjacent field site [27] , [34] , [43] , [49] . We therefore assessed the extent to which absolute CH 4 emissions and CH 4 emissions as a function of species composition (i.e. the key finding of our mesocosm experiments) differ between mesocosms and field plots of the adjacent marsh. Mean growing season CH 4 emissions were quantified in the Salt Marsh Accretion Response to Temperature eXperiment (SMARTX) operating in a high elevation, Spartina -dominated area and a low elevation, Schoenoplectus -dominated area of the adjacent marsh. A detailed description of the SMARTX study design is given by Noyce et al. [56] . Here we do not analyze temperature effects on CH 4 emissions, but compare CH 4 emissions from the ambient plots of the two plant communities ( n = 3) and assess the relationship between the relative abundance of the two plant species and CH 4 emissions across all treatments ( n = 24). Measurements CH 4 emission measurements followed the flux measurement protocol for marsh organs presented in Mueller et al. [50] with slight modifications for CH 4 . In July 2011, in the second consecutive growing season of Experiment 1, mesocosms were carefully moved from the marsh organs into 120-L containers positioned directly adjacent. Due to poor plant survival at the lowest elevations, CH 4 emission measurements were restricted to elevations of MSL −5 cm and higher. Containers were filled with creek water to the depth that corresponded to the water level that mesocosms were last exposed to in the marsh organ. Clear, acrylic flux chambers (volume = 7.5 L) were placed onto each mesocosm and sealed. Gas samples (20 mL) were collected from the chamber headspace every 20 min for a period of 2 h and analyzed for CH 4 using a gas chromatograph (Varian 450, Agilent Technologies). CH 4 fluxes were calculated from linear regression slopes (chamber headspace [CH 4 ] vs. time) following the ideal gas law, using chamber temperature for each given time point and assuming ambient pressure. Only fluxes with R 2 ≥ 0.8 were used (mean R 2 = 0.95 ± 0.05 SD, N = 82). The detection limit was 9 µmol CH 4 m −2 h −1 . CH 4 emission measurements of Experiment 2 were conducted in Sep 2012, after c. 4 months of plant growth in the marsh organ in the first growing season of the experiment. Sampling procedures followed Experiment 1, with the exception that samples were analyzed using a Shimadzu GC-14A (Shimadzu Corporation). Only fluxes with R 2 ≥ 0.8 were used (mean R 2 = 0.96 ± 0.05 SD, N = 16). The detection limit was 2 µmol CH 4 m −2 h −1 . Spartina did not survive at MSL ±0 cm in Experiment 2. This elevation was therefore not considered for comparisons between species. Field CH 4 emission measurements in SMARTX were conducted monthly from Jun 12 to Sep 4, 2019, 3 years after flux chamber bases were installed. Chambers (40 × 40 × 40 cm) were stacked onto each chamber base (total volume = 64–256 L) and covered with an opaque shroud. An ultra-portable greenhouse-gas analyzer (Los Gatos Research) was used to measure headspace CH 4 concentrations every 3 s for 5 min. Fluxes were calculated as described above and only fluxes that were significant at p ≤ 0.05 were included in the analysis. Detection limit was <0.6 µmol CH 4 m −2 h −1 . In order to gain more mechanistic insight into potential effects of plant species shifts on CH 4 dynamics, soil redox conditions were measured in Experiment 2. Redox measurements were conducted during a single campaign in Sep 2012, after c. 4 months of plant growth in the marsh organ. Measurements were taken on n = 3 mesocosms per plant species and elevation at low tide. Three platinum-tipped redox electrodes [57] were inserted to a soil depth of 10 cm and allowed to equilibrate for 45 min. For readings, a calomel reference electrode (Fisher Scientific accumet) was inserted to a soil depth of 1 cm, and reference and redox electrodes were connected to a portable conductivity meter (Fisher Scientific accumet). Readings were corrected to the redox potential of the standard hydrogen electrode (+244 mV). Statistical analyses Analyses for Experiment 1 followed Langley et al. [27] . Three-way split-plot ANOVA was used to test for the effects of elevation (relative sea level), CO 2 , nitrogen, and their factorial interactions on CH 4 emissions. Marsh organ (1–6) was included as a random factor in the model. Within single marsh organs, mesocosms of the same treatment combination were considered technical duplicates, and the mean of each duplicate was considered the experimental unit. Replication was therefore n = 3 per treatment. Subsequent two-way ANOVAs were used to assess CO 2 and nitrogen effects within each elevation treatment. Linear and nonlinear regression analysis was used to further explore the relationship of elevation and CH 4 emissions. In order to identify possible relationships between plant biomass parameters and CH 4 emissions, we used biomass data obtained from a destructive harvest in Sep 2011 (c. two months after the CH 4 emission measurements) that has been presented in Langley et al. [27] . Specifically, we conducted linear regression to test whether biomass parameters (Supplementary Table 2) and CH 4 emissions are related both across and within various treatment combinations. Two-way ANOVA was used to test for effects of plant species and elevation on CH 4 emissions and soil redox in Experiment 2. Tukey’s HSD tests were used for pairwise comparisons following ANOVAs where appropriate. One-way ANOVA and linear regression were used to analyze the field CH 4 emission data (Fig. 4 ). CH 4 emission data typically show a log-normal distribution [40] , [58] . Data were log-transformed to improve normality (if required based on visual assessments) or when Levene’s test indicated heterogenous variance. Regression analyses were conducted with both log-transformed and untransformed data. Analyses were conducted using R version 3.5.2 (R Foundation for Statistical Computing) and PAST version 3.20. [59] . Reporting summary Further information on research design is available in the Nature Research Reporting Summary linked to this article.